FCA mediates thermal adaptation of stem growth by attenuating auxin action inArabidopsis Global warming is predicted to profoundly affect plant distribution and crop yield in the near future. Higher ambient temperature can influence diverse aspects of plant growth and development. In Arabidopsis , the basic helix-loop-helix transcription factor PHYTOCHROME-INTERACTING FACTOR 4 (PIF4) regulates temperature-induced adaptive responses by modulating auxin biosynthesis. At high temperature, PIF4 directly activates expression of YUCCA8 ( YUC8 ), a gene encoding an auxin biosynthetic enzyme, resulting in auxin accumulation. Here we demonstrate that the RNA-binding protein FCA attenuates PIF4 activity by inducing its dissociation from the YUC8 promoter at high temperature. At 28 °C, auxin content is elevated in FCA -deficient mutants that exhibit elongated stems but reduced in FCA -overexpressing plants that exhibit reduced stem growth. We propose that the FCA-mediated regulation of YUC8 expression tunes down PIF4-induced architectural changes to achieve thermal adaptation of stem growth at high ambient temperature. Plants adapt to high ambient temperature by adjusting plant architecture, such as elongation of hypocotyl and leaf stem and increase of leaf hyponasty [1] . These architectural adaptations help plants minimize the chance of heat damage and enhance evaporative leaf cooling for optimized plant growth [2] . However, a trade-off occurs when plants obtain the fitness benefits during long-term exposure to high temperature: plants having abnormally elongated stems tend to fall down and suffer from physiological imbalance [3] . This necessitates that there should be a fine-tuning mechanism that attenuates the effects of high temperature on stem growth. The Arabidopsis basic helix-loop-helix transcription factor PHYTOCHROME-INTERACTING FACTOR 4 (PIF4) plays a major role in high-temperature-induced plant responses. Elongation of hypocotyl, increase of hyponasty and induction of flowering are suppressed by pif4 mutations under high temperature conditions [1] , [4] , [5] . It has been reported that PIF4 directly regulates transcription of auxin biosynthesis enzyme genes, such as YUCCA8 ( YUC8 ), resulting in accumulation of auxin content [5] . PIF4 function is enhanced at high temperature. The PIF4 transcription is induced by exposure to high temperature [5] , [6] . In addition, protein stability and DNA-binding affinity of PIF4 are elevated at high ambient temperatures [6] , [7] . While the role of PIF4 in thermal regulation of stem growth is evident, it is not fully understood how PIF4 function is modulated at the molecular level. The Arabidopsis RNA-binding protein FCA is a critical component of the autonomous flowering pathway, which induces flowering by suppressing the floral repressor FLOWERING LOCUS C ( FLC ) [8] , [9] . FCA plays a role in alternative polyadenylation of its own pre-mRNA and antisense FLC RNA [8] , [10] . FCA also acts as a chromatin remodelling factor: it mediates histone demethylation of FLC chromatin, causing suppression of FLC expression [9] . Notably, it has been reported that FCA incorporates ambient temperature signals into the thermosensory flowering pathway [11] , raising a possibility that FCA would participate in plant responses to changes in ambient temperature. In this work, we demonstrate that FCA mediates the dissociation of PIF4 from its target gene chromatin, such as YUC8 , at high ambient temperature. FCA is recruited to YUC8 promoter through interaction with PIF4, resulting in the dissociation of PIF4 from YUC8 promoter and the suppression of YUC8 transcription. These observations illustrate that FCA attenuates PIF4 action in auxin accumulation occurring during high-temperature-induced stem growth to maintain architectural and physiological balance. FCA mediates thermal acceleration of stem growth While working on the role of FCA in thermosensory flowering, we found that FCA -deficient mutants fca-9 and fca-11 exhibited elongated hypocotyls at 28 °C compared with those of wild-type (Col-0) plants ( Fig. 1a ). In contrast, FCA -overexpressing transgenic plants ( 35S:FCA ) had shorter hypocotyls under identical conditions, suggesting that FCA is associated with ambient temperature regulation of hypocotyl growth. 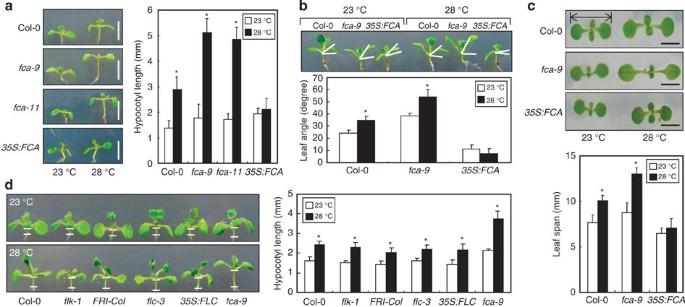Figure 1: FCA mediates the thermal acceleration of stem growth. Plants were grown on MS-agar plates at 23 °C under continuous light conditions for 4 days and further grown at either 23 or 28 °C for 3 days. Measurements of 15–20 seedlings were averaged and statistically treated using Studentt-test (*P<0.01). Bars indicate s.e. (a)fcamutants have elongated hypocotyls at 28 °C. (n=20). Scale bars, 1 cm. (b) Hyponasty increases infca-9at 28 °C. (n=15). (c) Leaf span is elongated infca-9at 28 °C. (n=20). Scale bars, 5 mm. (d) High-temperature-induced hypocotyl elongation offca-9is not related withFLC. (n=17). Figure 1: FCA mediates the thermal acceleration of stem growth. Plants were grown on MS-agar plates at 23 °C under continuous light conditions for 4 days and further grown at either 23 or 28 °C for 3 days. Measurements of 15–20 seedlings were averaged and statistically treated using Student t -test (* P <0.01). Bars indicate s.e. ( a ) fca mutants have elongated hypocotyls at 28 °C. ( n=20 ). Scale bars, 1 cm. ( b ) Hyponasty increases in fca-9 at 28 °C. ( n=15 ). ( c ) Leaf span is elongated in fca-9 at 28 °C. ( n=20 ). Scale bars, 5 mm. ( d ) High-temperature-induced hypocotyl elongation of fca-9 is not related with FLC . ( n=17 ). Full size image We also examined the effects of fca mutation on leaf hyponasty and leaf stem growth, which are also affected by high temperature [1] , [12] . Leaf hyponasty markedly increased in fca-9 when grown at 28 °C, but it was reduced in 35S:FCA transgenic plants ( Fig. 1b ). In addition, leaf stem (petiole) was elongated in fca-9 compared with that of Col-0 plants, but the high temperature sensitivity disappeared in 35S:FCA transgenic plants ( Fig. 1c ). These observations support the notion that FCA mediates the high ambient temperature-induced architectural modifications. FCA-mediated ambient temperature signals regulate flowering time via the floral repressor FLC [8] , [9] , [11] . To examine whether FLC is involved in the enhanced stem growth in fca-9 at high temperature, we measured hypocotyl growth in FLC -deficient flc-3 mutant and FLC -accumulating plants, such as flk-1 and fld-6 mutants [13] , [14] , active FRIGIDA ( FRI ) allele-containing FRI -Col plants [15] and FLC -overexpressing plants. Their hypocotyl growth was similar to that of Col-0 plants at 28 °C ( Fig. 1d , Supplementary Fig. 1 ), showing that the accelerated hypocotyl elongation in fca-9 at 28 °C is not related with FLC . IAA content is elevated in fca-9 at 28 °C To obtain clues as to how FCA regulates stem growth at high temperature, we investigated the expression of genes encoding biosynthetic enzymes of ethylene, gibberellic acid, brassinosteriod and auxin, which mediate stem growth [16] , [17] . Among those, only auxin biosynthetic enzyme genes were significantly induced in fca-9 when grown at 28 °C ( Supplementary Fig. 2 ). Among the INDOLE-3-ACETIC ACID INDUCIBLE ( IAA ) and YUC genes tested, IAA29 and YUC8 , which have been shown to mediate high-temperature-induced stem elongation [1] , [5] , were induced by more than sixfold in the high-temperature-treated fca-9 mutant ( Fig. 2a,b ). Auxin-responsive SMALL AUXIN UPREGULATED 20 ( SAUR20 ) and SAUR22 genes are also involved in high-temperature regulation of hypocotyl growth [4] . We found that they were expressed at higher levels in fca-9 compared with that in Col-0 plants at 23 °C ( Fig. 2c ), and their transcripts levels were further elevated in the high-temperature-treated fca-9 mutant. 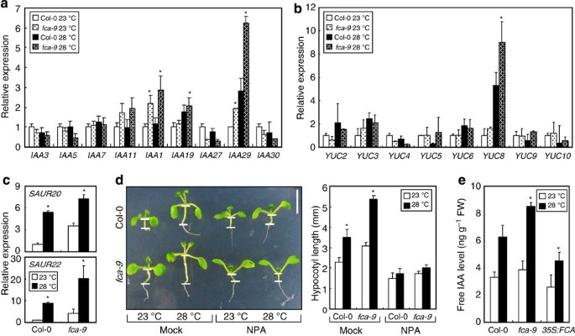Figure 2: IAA content is elevated infca-9at 28 °C. Transcript levels were measured by RT-qPCR. Biological triplicates were averaged and statistically treated using Student’st-test (*P<0.01). Bars indicate s.e. (a) Transcript levels ofIAAgenes infca-9. Plants were grown on MS-agar plates for 6 days at 23 °C and exposed to 28 °C for 24 h before harvesting whole plant materials. (b) Transcript levels ofYUCgenes infca-9. Total RNA samples prepared inawere used for RT–qPCR. (c) Transcript levels ofSAURgenes infca-9. Total RNA samples prepared inawere used for RT–qPCR. (d) Elongated hypocotyls offca-9is compromised in the presence of 100 μM 1-N-naphthylphthalamic acid (NPA). Plants were grown as described inFig. 1but in the presence of the auxin transport inhibitor NPA (left panel). Measurements of 20 hypocotyls were averaged and statistically treated using Student’st-test (*P<0.01; right panel). (e) Measurements of free IAA content infca-9. Plants were grown as described ina. Figure 2: IAA content is elevated in fca-9 at 28 °C. Transcript levels were measured by RT-qPCR. Biological triplicates were averaged and statistically treated using Student’s t -test (* P <0.01). Bars indicate s.e. ( a ) Transcript levels of IAA genes in fca-9 . Plants were grown on MS-agar plates for 6 days at 23 °C and exposed to 28 °C for 24 h before harvesting whole plant materials. ( b ) Transcript levels of YUC genes in fca-9 . Total RNA samples prepared in a were used for RT–qPCR. ( c ) Transcript levels of SAUR genes in fca-9 . Total RNA samples prepared in a were used for RT–qPCR. ( d ) Elongated hypocotyls of fca-9 is compromised in the presence of 100 μM 1- N -naphthylphthalamic acid (NPA). Plants were grown as described in Fig. 1 but in the presence of the auxin transport inhibitor NPA (left panel). Measurements of 20 hypocotyls were averaged and statistically treated using Student’s t -test (* P <0.01; right panel). ( e ) Measurements of free IAA content in fca-9 . Plants were grown as described in a . Full size image The upregulation of IAA29 , YUC8 and SAUR genes in fca-9 at 28 °C suggested that endogenous auxin content is elevated in fca-9 . To examine whether the elongated hypocotyl of fca-9 at 28 °C is caused by elevated auxin content, the mutant was grown at either 23 or 28 °C in the presence of the auxin transport inhibitor 1- N -naphthylphthalamic acid [18] . The high-temperature-induced hypocotyl elongation of the mutant was completely suppressed by 1- N -naphthylphthalamic acid ( Fig. 2d ). Direct measurements of IAA content revealed that at 28 °C, the level of free IAA was higher by 36% in fca-9 but lower by 28% in 35S:FCA transgenic plants compared with those in Col-0 plant ( Fig. 2e ), indicating that the high-temperature-induced hypocotyl elongation is due to elevated IAA content in fca-9 . FCA interacts with PIF4 in thermal induction of stem growth IAA29 , SAUR20, SAUR22 and YUC8 genes are regulated by PIF4 at a high temperature [1] , [4] , [5] , suggesting that PIF4 plays a role in the induction of the auxin-responsive genes in fca-9 . We first examined whether FCA interacts with PIF4. Bimolecular fluorescence complementation (BiFC) assays showed that they interact with each other in the nucleus ( Fig. 3a , Supplementary Fig. 3 ). in vitro pull-down assays also supported the physical association between FCA and PIF4 ( Fig. 3b ). 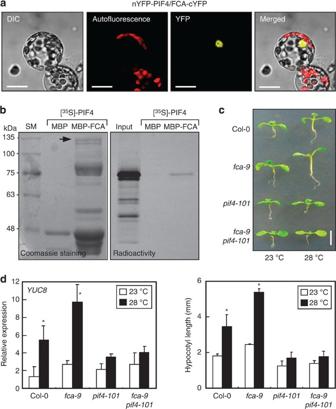Figure 3: FCA interacts with PIF4. (a) BiFC assays on FCA–PIF4 interaction. nYFP-PIF4 and cYFP-FCA gene fusions were coexpressed transiently inArabidopsisprotoplasts. FCA–PIF4 interactions were visualized by differential interference contrast microscopy. Scale bars, 10 μm. (b)In vitropull-down assays on FCA–PIF4 interaction. Recombinant MBP–FCA fusion protein was produced inE. colicells.35S-labelled PIF4 protein was prepared byin vitrotranslation. MBP alone was used as negative control (right panel). Part of Coomassie blue-stained gel was shown as loading control (left panel). (c) Hypocotyl growth offca-9 pif4-101. Plants grown on MS-agar plates for 4 days at 23 °C were further grown at 28 °C for 3 days (upper panel). Scale bar, 0.5 cm. Measurements of 15 hypocotyls were averaged and statistically treated using Student’st-test (*P<0.01; lower panel). Bars indicate s.e. (d) Transcript levels ofYUC8gene infca-9 pif4-101. Transcript levels were measured as described inFig. 2. Biological triplicates were averaged and statistically treated using Student’st-test (*P<0.01). Bars indicate s.e. Figure 3: FCA interacts with PIF4. ( a ) BiFC assays on FCA–PIF4 interaction. nYFP-PIF4 and cYFP-FCA gene fusions were coexpressed transiently in Arabidopsis protoplasts. FCA–PIF4 interactions were visualized by differential interference contrast microscopy. Scale bars, 10 μm. ( b ) In vitro pull-down assays on FCA–PIF4 interaction. Recombinant MBP–FCA fusion protein was produced in E. coli cells. 35 S-labelled PIF4 protein was prepared by in vitro translation. MBP alone was used as negative control (right panel). Part of Coomassie blue-stained gel was shown as loading control (left panel). ( c ) Hypocotyl growth of fca-9 pif4-101 . Plants grown on MS-agar plates for 4 days at 23 °C were further grown at 28 °C for 3 days (upper panel). Scale bar, 0.5 cm. Measurements of 15 hypocotyls were averaged and statistically treated using Student’s t -test (* P <0.01; lower panel). Bars indicate s.e. ( d ) Transcript levels of YUC8 gene in fca-9 pif4-101 . Transcript levels were measured as described in Fig. 2 . Biological triplicates were averaged and statistically treated using Student’s t -test (* P <0.01). Bars indicate s.e. Full size image We next explored the functional relationship between FCA and PIF4. A PIF4 -deficient pif4-101 mutant was crossed with fca-9 , resulting fca-9 pif4-101 . The high-temperature-induced hypocotyl elongation phenotype of fca-9 was suppressed in fca-9 pif4-101 , which is similar to the hypocotyl phenotype of pif4-101 ( Fig. 3c , Supplementary Fig. 4 ). In addition, the inductive effects of high temperature on YUC8 transcription were not observed in fca-9 pif4-101 and pif4-101 ( Fig. 3d ). Together with the elevated IAA content in fca-9 , these observations indicate that FCA is associated with the PIF4-regulated auxin biosynthesis. FCA regulates PIF4 binding to YUC8 chromatin A question was how FCA regulates PIF4 function. PIF4 gene is induced when plants grown at 16 °C are exposed to 28 °C (ref. 6 ). We examined whether the high-temperature induction of PIF4 gene is regulated by FCA. The inductive effects of high temperature on PIF4 transcription were still evident in fca-9 ( Supplementary Fig. 5 ). In addition, fca mutation did not affect the protein stability of PIF4 ( Supplementary Fig. 6 ). We next examined whether fca mutation influences the transcriptional activity of PIF4 using a β-glucuronidase (GUS) transient expression system in Arabidopsis protoplasts [19] , which were prepared from fca-9 mutant. It was found that the transcriptional activity of PIF4 was not altered in fca-9 , and coexpression of FCA did not affect the PIF4 activity ( Supplementary Fig. 7 ), indicating that FCA does not affect the transcriptional activity of PIF4. Instead, it was hypothesized that FCA might influence the DNA binding of PIF4. It has been known that PIF4 binds to G-box elements in YUC8 promoter, although it is unclear whether high temperature influences the DNA binding of PIF4 (ref. 5 ). Notably, it has recently been reported that PIF4 binds to FLOWERING LOCUS T ( FT ) promoter and its DNA binding is enhanced at high temperature [6] . We therefore hypothesized that FCA might influence the binding of PIF4 to YUC8 promoter in response to high temperature. Chromatin immunoprecipitation (ChIP) assays revealed that the binding of PIF4 to a sequence region covering G-box elements in YUC8 promoter, which was designated P2 region in this work ( Fig. 4a ), was elevated in both Col-0 and fca-9 plants exposed to 28 °C for 6 h ( Fig. 4b ). We next performed ChIP assays using plants that were exposed to 28 °C for longer time (24 h). Notably, while the binding of PIF4 to P2 was reduced to a basal level in Col-0 plants, the high-level binding of PIF4 to P2 was maintained in fca-9 ( Fig. 4c ). Consistent with these observations, the transcript levels of YUC8 were similar in Col-0 and fca-9 that were exposed to 28 °C for 6 h but was higher in fca-9 than in Col-0 when the plants were exposed to 28 °C for 24 h ( Fig. 4d ). It was therefore concluded that FCA does not affect the binding step of PIF4 to YUC8 promoter but trigger the dissociation of PIF4 from YUC8 promoter, especially under long-term exposure to high temperature. 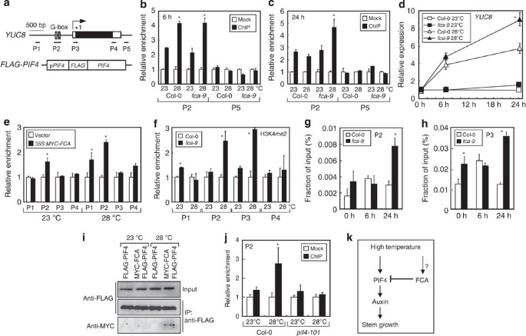Figure 4: FCA regulates PIF4 binding toYUC8promoter. Biological triplicates were averaged and statistically treated using Student’st-test (*P<0.01). Bars indicate s.e. (a) Genomic structure ofYUC8gene. P1 to P5 sequence regions were used in ChIP assays. Black boxes are exons, and white boxes are untranslated regions. The FLAG-PIF4 expression construct, in which a FLAG octapolypeptide-coding sequence is fused in-frame to the 5′ end ofPIF4gene under the control of the endogenousPIF4promoter consisting of approximately 2-kbp sequence upstream of the translation start site, is shown at the bottom. (b,c) ChIP assays on the effects of FCA on PIF4 binding toYUC8promoter. The FLAG-PIF4 gene fusion was transformed into Col-0 andfca-9plants. Plants grown on MS-agar plates for 6 days at 23 °C were further grown at either 23 or 28 °C for 6 h (b) and 24 h (c) before extracting chromatin from whole plants. ChIP assays were performed with P2 and P5 sequences using an anti-FLAG antibody. (d) Accumulation kinetics ofYUC8transcripts infca-9after 28 °C treatment. Transcript levels were measured as described inFig. 2. (e) ChIP assays on FCA binding toYUC8chromatin. A MYC-FCA fusion was overexpressed in Col-0 plants. Chromatin was prepared as described inc. ChIP assays were performed with P1 to P4 sequences using an anti-MYC antibody. (f) Histone modifications atYUC8chromatin infca-9. Plant growth and chromatin preparation were performed as described inc. ChIP assays were performed using an anti-H3K4me2 antibody. (g,h) Kinetics of histone modifications atYUC8chromatin infca-9. Chromatin was prepared from plants at different time points after exposure to 28 °C. ChIP assays were performed with either P2 (g) or P3 (h) sequence using an anti-H3K4me2 antibody. (i) Coimmunoprecipitation assays on FCA–PIF4 interaction. The FLAG-PIF4 expression construct was transformed into35S:MYC-FCAtransgenic plants. Plants were treated with 28 °C, as described inc. Imunoprecipitation (IP) was performed using an anti-FLAG antibody. Input represents 5% of the IP reaction. (j) ChIP assays on FCA binding toYUC8chromatin inpif4-101. The assays were performed as described in (c) usingpif4-101mutant overexpressing MYC-FCA driven by the CaMV 35S promoter. (k) FCA attenuation of PIF4 action in thermal acceleration of stem growth. FCA regulates the binding of PIF4 toYUC8promoter, providing an adaptation strategy at high temperature. Figure 4: FCA regulates PIF4 binding to YUC8 promoter. Biological triplicates were averaged and statistically treated using Student’s t -test (* P <0.01). Bars indicate s.e. ( a ) Genomic structure of YUC8 gene. P1 to P5 sequence regions were used in ChIP assays. Black boxes are exons, and white boxes are untranslated regions. The FLAG-PIF4 expression construct, in which a FLAG octapolypeptide-coding sequence is fused in-frame to the 5′ end of PIF4 gene under the control of the endogenous PIF4 promoter consisting of approximately 2-kbp sequence upstream of the translation start site, is shown at the bottom. ( b , c ) ChIP assays on the effects of FCA on PIF4 binding to YUC8 promoter. The FLAG-PIF4 gene fusion was transformed into Col-0 and fca-9 plants. Plants grown on MS-agar plates for 6 days at 23 °C were further grown at either 23 or 28 °C for 6 h ( b ) and 24 h ( c ) before extracting chromatin from whole plants. ChIP assays were performed with P2 and P5 sequences using an anti-FLAG antibody. ( d ) Accumulation kinetics of YUC8 transcripts in fca-9 after 28 °C treatment. Transcript levels were measured as described in Fig. 2 . ( e ) ChIP assays on FCA binding to YUC8 chromatin. A MYC-FCA fusion was overexpressed in Col-0 plants. Chromatin was prepared as described in c . ChIP assays were performed with P1 to P4 sequences using an anti-MYC antibody. ( f ) Histone modifications at YUC8 chromatin in fca-9 . Plant growth and chromatin preparation were performed as described in c . ChIP assays were performed using an anti-H3K4me2 antibody. ( g , h ) Kinetics of histone modifications at YUC8 chromatin in fca-9 . Chromatin was prepared from plants at different time points after exposure to 28 °C. ChIP assays were performed with either P2 ( g ) or P3 ( h ) sequence using an anti-H3K4me2 antibody. ( i ) Coimmunoprecipitation assays on FCA–PIF4 interaction. The FLAG-PIF4 expression construct was transformed into 35S : MYC-FCA transgenic plants. Plants were treated with 28 °C, as described in c . Imunoprecipitation (IP) was performed using an anti-FLAG antibody. Input represents 5% of the IP reaction. ( j ) ChIP assays on FCA binding to YUC8 chromatin in pif4-101 . The assays were performed as described in ( c ) using pif4-101 mutant overexpressing MYC-FCA driven by the CaMV 35S promoter. ( k ) FCA attenuation of PIF4 action in thermal acceleration of stem growth. FCA regulates the binding of PIF4 to YUC8 promoter, providing an adaptation strategy at high temperature. Full size image FCA induces chromatin modification at YUC8 FCA requires a histone demethylase, which targets the active marker histone-3 lysine-4 dimethylation (H3K4me2), to downregulate FLC expression [9] . We therefore suspected that FCA influences the dissociation of PIF4 from YUC8 promoter via chromatin remodelling. ChIP assays showed that FCA binds to P2 region in YUC8 chromatin at 23 °C and its DNA binding was considerably elevated at 28 °C ( Fig. 4e ). FCA also bound to P1 region, which is approximately 500 bases upstream of P2 region, at 28 °C. In addition, the levels of H3K4me2 was elevated by more than twofold in P2 region in fca-9 at 28 °C ( Fig. 4f ). The H3K4me2 level was also elevated in P3 region covering the transcription start site. These data suggest that FCA promotes the dissociation of PIF4 from the YUC8 promoter at 28 °C by modifying YUC8 chromatin. We next monitored the kinetics of H3K4me2 accumulation in fca-9 after exposure to 28 °C. In Col-0, the H3K4me2 level in the P2 region was elevated by approximately twofold at 6 h but reduced to a basal level at 24 h ( Fig. 4g ). In fca-9 , it was largely unchanged at 6 h but significantly elevated by more than twofold at 24 h. The kinetic patterns of H3K4me2 accumulation in P3 regions were similar to those observed in P2 regions of both Col-0 and fca-9 plants ( Fig. 4h ). We propose that FCA-mediated demethylation events are induced by long periods of exposure to high temperature. FCA modulates the dissociation of PIF4 from YUC8 chromatin A critical question was how high-temperature signals are incorporated into the FCA–PIF4-YUC8 module. FCA transcription was only moderately induced by approximately twofold at 28 °C ( Supplementary Fig. 8a ). In addition, high temperature did not discernibly affect the FCA protein stability ( Supplementary Fig. 8b ). We next performed coimmunoprecipitation assays on Col-0 plants coexpressing FLAG-PIF4 and MYC-FCA fusions using anti-FLAG and anti-MYC antibodies for the pull down of the fusion proteins. FCA interacted with PIF4 in planta primarily at 28 °C ( Fig. 4i , Supplementary Fig. 9 ). Furthermore, ChIP assays on pif4-101 mutant overexpressing MYC-FCA showed that FCA binding to YUC8 chromatin did not occur in the mutant at 28 °C ( Fig. 4j ). Together with the increased binding of PIF4 to YUC8 chromatin ( Fig. 4b ), these observations indicate that at high temperatures, PIF4 recruits FCA to the chromatin, where FCA induces chromatin modifications, causing PIF4 dissociation ( Supplementary Fig. 10 ). All together, we conclude that FCA tunes down the high-temperature-induced stem elongation by attenuating PIF4 action probably through remodelling of YUC8 chromatin ( Fig. 4k ). We found that FCA, which is otherwise a well-characterized RNA-binding protein functioning in flowering time control [8] , [9] , plays a role in modulating PIF4 induction of YUC8 in response to high temperature. On the basis of our data, we propose that the FCA-mediated counteracting mechanism is required to offset the accelerated stem elongation at high temperature within the ambient temperature range, contributing to thermal adaptation of stem growth. The physiological role of FCA in this high temperature signalling is similar to that proposed for HIGH EXPRESSION OF OSMOTICALLY RESPONSIVE GENES 1 (HOS1) E3 ubiquitin ligase. In cold acclimation signalling, HOS1 triggers protein degradation of INDUCER OF CBF EXPRESSION 1, which induces transcription of C-REPEAT BINDING FACTOR 1 and 3 (refs 20 , 21 ). The HOS1-mediated negative regulation of cold signalling is important for maintaining physiological balance under prolonged cold temperature conditions, because over-induction of cold response causes developmental defects and growth retardation [22] . It is notable that FLOWERING LOCUS D (FLD), which acts together with FCA to modify FLC chromatin [9] , is not functionally related with FCA in thermal regulation of hypocotyl growth. While our data strongly support the role of FCA in YUC8 chromatin modification at high temperature, the observed modification of YUC8 chromatin in fca -9 background would simply reflect the thermal induction of YUC8 in the mutant. Future work will be required to clarify this uncertainty concerning the molecular mechanism of FCA in the transcriptional control of YUC8 and its functional relevance in thermal regulation of hypocotyl growth. Plant materials and growth conditions All Arabidopsis thaliana lines used were in Columbia (Col-0) background. Plants were grown in a controlled culture room at 23 °C with relative humidity of 55% under continuous light conditions, unless specified otherwise, with white light illumination (120 μmol photons m −2 s −1 ) provided by fluorescent FLR40D/A tubes (Osram, Seoul, Korea). The fca-9 , fca-11 and pif4-101 mutants and 35S:FCA transgenic plants have been described previously [1] , [23] , [24] . To generate 35S:MYC-FCA transgenic plants, a full-size FCA γ cDNA was fused in-frame to the 3′ end of the MYC-coding sequence in the myc-pBA vector [25] . The expression construct was transformed into Col-0 plants. To examine the effects of high temperature on hypocotyl growth, leaf spanning and leaf hyponasty, plants grown on 1/2 × Murashige and Skoog-agar plates (MS-agar plates) at 23 °C for 4 days were further grown at either 23 or 28 °C for 3 additional days. Plants (15–20) were measured and averaged. To analyse the effects of high temperature on gene expression, plants grown at 23 °C for 6 days on MS-agar plates were further grown at either 23 or 28 °C for 24 h. Whole plants were used for the extraction of total RNA. Analysis of gene transcript levels Transcript levels were determined by reverse transcription-mediated quantitative real-time PCR (RT–qPCR). RT–qPCR reactions were carried out according to the guidelines that have been proposed to guarantee reproducible and accurate measurements [26] . Extraction of total RNA samples from appropriate plant materials and RT–PCR conditions have been described previously [27] . The RNA samples were pretreated extensively with RNase-free DNase to eliminate contaminating genomic DNA before use. RT–qPCR reactions were conducted in 96-well blocks with an Applied Biosystems 7500 Real-Time PCR System using the SYBR Green I master mix in a volume of 25 μl. The PCR primers were designed using the Primer Express Software installed into the system and listed in Supplementary Table 1 . The two-step thermal cycling profile employed was 15 s at 94 °C and 1 min at 68 °C. An eIF4A gene (At3g13920) was included in the reactions as internal control for normalizing the variations in cDNA amounts used. All RT-qPCR reactions were carried out in biological triplicates using RNA samples extracted from three independent plant materials grown under identical growth conditions. The comparative ΔΔ C T method was employed to evaluate relative quantities of each amplified product in the samples. The threshold cycle ( C T ) was automatically determined for each reaction by the system set with default parameters. The specificity of the PCR reactions was determined by melt curve analysis of the amplified products using the standard method installed in the system. Measurements of free IAA content Plants grown on MS-agar plates at 23 °C for 6 days were incubated at 28 °C for 24 h. Aerial plants parts were harvested for the extraction of free IAA. Plant materials were finely ground in liquid nitrogen, and 0.1 g of the powder was extracted in 1 ml of ethyl acetate-formic acid solution (99.5:0.5) containing 20 ng of D 5 -IAA as a standard. The samples were then vortex mixed for 10 min and centrifuged at 16,000 g for 20 min at 4 °C. The supernatants were then evaporated at room temperature in SpeedVac (Eppendorf, Hamburg, Germany). The pellets were resuspended in 50 μl of methanol–water solution (70:30) and dissolved for 5 min using an ultrasonic bath (Branson, Danbury, CT). IAA content was measured using liquid chromatography (Agilent Technologies, Santa Clara, CA), which was coupled to a mass spectrometer (Applied Biosystems, Foster City, CA), as described previously [28] . Separation was performed on a Zorbax Eclipse column (Agilent technologies). Mobile phases A (0.05% acetic acid in water) and B (0.05% acetic acid in acetonitrile) were used for the separation. The mass spectrometer was operated in the positive ionization mode with an ion spray voltage of 5,500 V and a turbo gas temperature of 700 °C. BiFC assay BiFC assays were carried out as described previously [29] . A full-size FCA gene was fused in-frame to the 3′ end of a DNA sequence encoding the carboxyl-terminal half of yellow fluorescent protein (YFP) in the pSATN-cYFP-C1 vector (E3082). A PIF4 cDNA was fused in-frame to the 3′ end of a DNA sequence encoding the amino-terminal half of YFP in the pSATN-nYFP-C1 vector (E3081). The expression constructs were co-transformed into Arabidopsis protoplasts. The expression of the fusion constructs was visualized by differential interference contrast microscopy and fluorescence microscopy using a Zeiss LSM510 confocal microscope (Carl Zeiss, Yena, Germany). Reconstitution of YFP fluorescence was observed using a confocal microscope with the following YFP filter set up: excitation 515 nm, 458/514 dichroic, and emission 560–615 nm BP filter. Preparation of MBP–FCA fusion protein The FCA gene was subcloned into the pMAL-c2X Escherichia coli expression vector (NEB, Ipswich, MA) containing a maltose-binding protein (MBP)-coding sequence. Recombinant MBP and MBP–FCA fusion proteins were produced in E. coli Rosetta2 (DE3) pLysS strain (Novagen, Madison, WI) and purified as described previously [29] . One-tenth volume of precultured cells (5 ml) was added to 500 ml of Luria-Bertani medium and cultured at 37 °C until OD 600 =0.3–0.6. Then, isopropyl-β- D -thiogalactopyranoside was added to the culture at a final concentration of 0.5 mM, and the mixture was incubated for 16 h at 22 °C to induce protein production. Cells were harvested and resuspended in MBP buffer (20 mM Tris-HCl, pH 7.4, 200 mM NaCl, 1 mM EDTA, 10 mM 2-mercaptoethanol, 1 mM phenylmethylsulfonyl fluoride (PMSF) and protease inhibitor cocktail (Sigma-Aldrich, St Louis, MO; Cat No. P9599)). Cell lysates were prepared by three cycles of freezing and thawing followed by centrifugation. The supernatants were stored at −80 °C until use. In vitro pull-down assay To examine the interactions of FCA with PIF4, the PIF4 cDNA was amplified by RT–PCR and subcloned into the pGBKT7 vector, which contains the T7 RNA polymerase promoter upstream of a multiple cloning sequence. The [ 35 S]methionine-labelled PIF4 protein was synthesized by in vitro translation using the TNT coupled reticulocyte lysate system (Promega, Madison, WI). Five μl of the 35 S-labelled protein solution was incubated with 1 μg of purified MBP or MBP–FCA fusion protein bound to MBP beads in 1 ml of binding buffer (50 mM Tris-HCl, pH 8.0, 100 mM NaCl, 10% glycerol, 1% Triton-X-100, 1 mM PMSF and protease inhibitor cocktail (Sigma-Aldrich)) containing 5% skim milk for 12 h at 4 °C. The beads were washed 10 times with TN buffer (25 mM Tris-HCl, pH 8.0, 100 mM NaCl). The bound proteins were eluted with 1 × SDS-polyacrylamide gel electrophoresis loading buffer by heating for 10 min at 70 °C and subject to SDS-polyacrylamide gel electrophoresis and autoradiography. ChIP assay ChIP assays were performed as described previously [30] . The assays were performed in biological triplicates using three independent plant materials grown under identical growth conditions. Plants were grown on MS-agar plates for 6 days and further grown for appropriate time periods at either 23 or 28 °C. Whole plants were harvested for the analysis. Plant materials were vacuum infiltrated with 1% (v/v) formaldehyde for cross-linking and ground in liquid nitrogen after quenching the cross-linking process. The ground powder was resuspended in nuclear extraction buffer (1.7 M sucrose, 10 mM Tris-Cl, pH 7.5, 2 mM MgCl 2 , 0.15% Triton-X-100, 5 mM β-mercaptoethanol, 0.1 mM PMSF and protease inhibitor cocktail tablets (Sigma-Aldrich)) and centrifuged at 16,000 g for 1 h at 4 °C to obtain nuclear fraction. The nuclear fraction was lysed with lysis buffer (50 mM Tris-Cl, pH 8.0, 0.5 M EDTA, 1% SDS and protease inhibitor cocktail tablets (Sigma-Aldrich)) to extract chromatin. Chromatin preparations were sonicated into 0.4–0.7-kb fragments. Five μg of anti-MYC (Millipore, Billerica, MA; Cat No. 05-724), anti-FLAG (Sigma-Aldrich; Cat No. F1804) or anti-H3K4me2 (Millipore; Cat No. 05-1338) antibody was added to the chromatin solutions, which were precleared with salmon sperm DNA/ Protein G agarose beads (Roche, Indianapolis, IN). The precipitates were eluted from the beads. Cross-links were reversed, and residual proteins were removed by incubation with proteinase K. DNA was recovered using the Promega spin column (Promega). Quantitative PCR was used to determine the amounts of genomic DNA enriched in the chromatin preparations, and the values were normalized to the amount of input in each sample. The primers used are listed in Supplementary Table 1 . Coimmunoprecipitation assay Coimmunoprecipitation assays were performed as described previously [31] . Plants were grown for 6 days at 23 °C and further grown for 24 h at either 23 or 28 °C. Whole plants were harvested for the assays. Plant materials were ground in liquid nitrogen and proteins were extracted in coimmunoprecipitation buffer (50 mM Tris-Cl pH 7.4, 500 mM NaCl, 10% glycerol, 5 mM EDTA, 1% Triton-X-100, 1% Nonidet P-40 and protease inhibitor cocktail tablets (Sigma-Aldrich)). Extract (5%) was used as the input control. Five μg of anti-FLAG antibody (Sigma-Aldrich; Cat No. F1804) was added to the extract and incubated for 2 h. After the incubation, protein G agarose beads were added and further incubated for 2 h. The beads were then washed five times with coimmunoprecipitation buffer lacking protease inhibitor cocktail. To elute proteins, 50 μl of 2 × SDS loading buffer (100 mM Tris-Cl pH 6.8, 4% sodium dodecyl sulfate, 0.2% bromophenol blue, 20% glycerol, 200 mM DTT) was added to the beads and incubated at 100 °C for 10 min. Eluted proteins (20%) was used for IP control. Anti-FLAG antibody (Sigma-Aldrich; Cat No. F1804) and anti-MYC antibody (Millipore; Cat No. 05-724) were used for the detection of FLAG-PIF4 and MYC-FCA, respectively (dilution=1:4,000). Uncropped blot images of Fig. 4i are shown in Supplementary Fig. 11 . How to cite this article: Lee, H.-J. et al. FCA mediates thermal adaptation of stem growth by attenuating auxin action in Arabidopsis . Nat. Commun. 5:5473 doi: 10.1038/ncomms6473 (2014).